The tiger genome and comparative analysis with lion and snow leopard genomes Tigers and their close relatives ( Panthera ) are some of the world’s most endangered species. Here we report the de novo assembly of an Amur tiger whole-genome sequence as well as the genomic sequences of a white Bengal tiger, African lion, white African lion and snow leopard. Through comparative genetic analyses of these genomes, we find genetic signatures that may reflect molecular adaptations consistent with the big cats’ hypercarnivorous diet and muscle strength. We report a snow leopard-specific genetic determinant in EGLN1 (Met39>Lys39), which is likely to be associated with adaptation to high altitude. We also detect a TYR 260G>A mutation likely responsible for the white lion coat colour. Tiger and cat genomes show similar repeat composition and an appreciably conserved synteny. Genomic data from the five big cats provide an invaluable resource for resolving easily identifiable phenotypes evident in very close, but distinct, species. The tiger ( Panthera tigris ), the largest felid species on Earth and a widely recognized symbol for wildlife conservation [1] , is one of the world’s most endangered species. Tigers are a keystone species and natural indicators of the health of the ecological communities in which they are found [2] . The current estimates of wild tigers range from just 3,050 to 3,950 individuals. It is postulated that without conservation measures tigers will soon become extinct in the wild, thus turning the preservation of existing wild tiger populations into a major goal of conservation efforts [3] , [4] . Tigers comprise of nine genetically validated subspecies [1] , [5] , [6] . Four of these went extinct in the wild during the last century (Javan, Balinese, South China and Caspian tigers), leaving five extant subspecies (Amur, Bengal, Indochinese, Malayan and Sumatran tigers) [5] . The Amur tiger ( Panthera tigris altaica ) is the largest in overall size and the only subspecies inhabiting snow-covered regions. Previous genetic studies using mitochondrial and nuclear loci have helped to elucidate the phylogeography and population genetics of tigers [1] , [5] , [6] , [7] , and the low coverage genome (1.8 × ) of the domestic cat ( Felis catus ) has provided insights into felid evolution [8] , [9] . However, no whole-genome reference sequence has been reported for the tiger, or any of the Panthera species, thus limiting current understanding of genetic diversity and demography [10] , [11] , [12] . We report the first tiger genome sequence assembly and annotation as well as a comparative analysis of the lion ( Panthera leo ) and snow leopard ( Panthera uncia ) genomes. We describe genotypic variation and genotype association analyses with species-specific phenotypes and adaptation. Panthera whole-genome sequences provide valuable information on genome organization, evolutionary divergence and overall endemic diversity. The Amur tiger genome The DNA of a 9-year-old male Amur tiger from Everland Zoo in Korea was sequenced by Illumina HiSeq2000 ( Supplementary Fig. S1 , Supplementary Tables S1–S3 ). 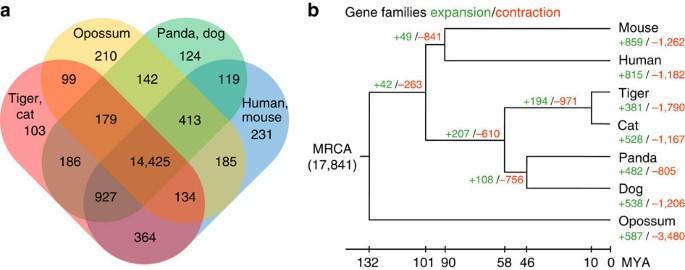Figure 1: Relationship of the tiger to other mammalian species. (a) Orthologous gene clusters in mammalian species. The Venn diagram shows the number of unique and shared gene families among seven mammalian genomes. (b) Gene expansion or contraction in the tiger genome. Numbers designate the number of gene families that have expanded (green, +) and contracted (red, −) after the split from the common ancestor. The most recent common ancestor (MRCA) has 17,841 gene families. The time lines indicate divergence times among the species. Sequence reads were assembled using SOAPdenovo [13] into scaffolds (2.4 Gb in length) having an N50 length of 8.84 Mb (contig N50 length of 29.8 kb; Table 1 , Supplementary Figs S2–S4 , Supplementary Tables S4 and S5 , Methods ). Assembly quality was assessed by aligning the assembled tiger blood transcripts and cat EST sequences onto the tiger scaffolds (>96% coverage and 98.9% mapping rate, respectively), and heterozygous single nucleotide variants (SNVs) were validated by the Sanger method ( Supplementary Tables S6–S9 , Supplementary Methods ). Additionally, analysis of the tiger draft genome assembly for core eukaryotic genes [14] revealed homologues for >93.4% of conserved genes in the assembly ( Supplementary Table S10 ). The tiger genome sequence shows 95.6% similarity to the domestic cat ( Supplementary Table S11 ) from which it diverged approximately 10.8 million years ago (MYA) [15] ; human and gorilla have 94.8% similarity and diverged around 8.8 MYA (from TimeTree). This high similarity allowed us to improve the assembly of the tiger genome by using the recently completed high coverage (12 × coverage) domestic cat genome ( Supplementary Fig. S5 , Supplementary Tables S12–S17 , Supplementary Methods ). For comparative genomic analysis of big cats, we also sequenced four other Panthera genomes ( Table 1 , Supplementary Tables S1 and S18 ): a white Bengal tiger ( Panthera tigris tigris ), an African lion, a white African lion and a snow leopard; their genome sequences were aligned with the domestic cat and tiger genomes. Table 1 Global statistics of the Panthera genomes. Full size table Adaptation of the big cats The assembled Amur tiger genome was predicted to contain 20,226 protein-coding genes ( Supplementary Tables S19–S23 , Supplementary Methods ) and 2,935 non-coding RNAs ( Supplementary Table S24 , Supplementary Methods ). To create a detailed annotation of the tiger proteome, gene clusters were constructed using seven mammalian genomes (tiger, cat, human, dog, mouse, giant panda and opossum). The tiger proteome contained 14,954 orthologous gene families. Among these, 14,425 orthologous gene families were shared by all seven genomes, whereas 103 orthologous gene families were exclusively shared by the tiger and cat ( Fig. 1a , Supplementary Fig. S6 , Supplementary Table S25 ). The Felidae-specific gene families contained 287 InterPro domains ( Supplementary Tables S26–S29 ). Based on the comparison of orthologous gene families among seven mammalian species, the Amur tiger genome displays 381 expanded and 1,790 contracted gene families compared with the feline common ancestor ( Fig. 1b , Supplementary Figs S7 and S8 ). The tiger genome is particularly enriched in olfactory receptor activity (GO:0004984, P =5.75 × 10 −185 , ChiSquare test followed by a Fisher's exact test, 289 genes), G-protein coupled receptor signalling pathway (GO:0007186, P =2.98 × 10 −106 , 302 genes), signal transducer activity (GO:0004871, P =2.25 × 10 −74 , 295 genes), amino-acid transport (GO:0006865, P =3.09 × 10 −10 , 16 genes) and protein metabolic process (GO:0019538, P =5.72 × 10 −10 , 220 genes) ( Supplementary Fig. S9 , Supplementary Table S30 ). In most cats, smell has an important role in social behaviour such as territory ownership and mating, while vision and hearing are important for hunting [16] . Figure 1: Relationship of the tiger to other mammalian species. ( a ) Orthologous gene clusters in mammalian species. The Venn diagram shows the number of unique and shared gene families among seven mammalian genomes. ( b ) Gene expansion or contraction in the tiger genome. Numbers designate the number of gene families that have expanded (green, +) and contracted (red, −) after the split from the common ancestor. The most recent common ancestor (MRCA) has 17,841 gene families. The time lines indicate divergence times among the species. Full size image Additionally, we investigated Panthera lineage-specific amino-acid changes by comparison with the known genes from the human, dog and mouse. A total of 3,646 genes had amino-acid changes specific to big cats (Amur tiger, white tiger, snow leopard, African lion and white lion; Supplementary Tables S31 and S32 ), and 5,882 genes had amino-acid changes unique to the felid lineage (big cats plus domestic cat). Among these, 1,376 genes had big cat-specific amino-acid changes that were found to be protein functional changes according to computational predictions (PolyPhen2 [17] ). Metabolism pathways associated with protein and fatty acid, which are important sources of energy, were enriched with genes having Panthera -specific functional changes; histidine metabolism ( P =0.00024, Fisher's exact test, six genes), beta-alanine metabolism ( P =0.00078, six genes), phenylalanine metabolism ( P =0.014, three genes), valine, leucine and isoleucine degradation ( P =0.035, six genes), cysteine and methionine metabolism ( P =0.037, four genes), fatty acid metabolism ( P =0.00038, eight genes) and fat digestion and absorption ( P =0.025, five genes) ( Supplementary Tables S33 and S34 ). These signals of amino-acid metabolism have been associated with an obligatory carnivorous diet [18] . In order to detect tiger genes evolving under positive selection, we used the conserved genome synteny methodology [19] (between human and other mammalian species (cat, dog, mouse and panda)) and a branch-site likelihood ratio test (Methods). A total of 178 positively selected genes out of 7,415 high-quality ortholog genes were identified in the Amur tiger ( Supplementary Table S35 , Supplementary Data 1 ). Functional categories for positively selected genes were over-represented in muscle filament sliding (GO:0030049, P =0.0049, Fisher's exact test, MYH7 , TPM4 and TNNC2 ), filamentous actin (GO:0031941, P =0.0062, TPM4 and MYO1A ) and stress fibre (GO:0001725, P =0.0039, MYH7 , TPM4 and ACTN4 ) ( Supplementary Table S36 , Supplementary Data 2 ). We also identified GO categories, which are evolving under significantly high constraints [19] ( Supplementary Tables S37–S39 , Supplementary Methods ). Significantly altered Ka / Ks ratios of non-synonymous to synonymous substitutions for GO categories ( P <0.01, Binomial test) revealed evidence of rapid evolution in the tiger for muscle strength (muscle contraction and actin cytoskeleton), energy metabolism (GTPase activity, ATP binding and energy reserve metabolic process), and sensory nerves (G-protein coupled receptor activity, olfactory receptor activity, visual perception and nervous system development) ( Supplementary Tables S40–S43 ). Genetic landscape of the snow leopard and white lion In addition to the Amur tiger data, we used sequence data from the four other big cats to investigate the genetic basis of several unique physiological or phenotypic traits. Snow leopards generally live in alpine areas, 3,350–6,700 m above sea level, in Central Asia [20] . Recent genome-wide association studies implicated two human loci EGLN1 (Egl nine homologue 1) and EPAS1 (endothelial PAS domain-containing protein 1) as mediating high-altitude adaptation [21] . We examined mutational substitutions in mammalian EGLN1 and EPAS1 genes and found that the snow leopard had unique amino-acid changes in both genes that were not found in other mammalian species. Although EGLN1 is highly conserved in mammals, Met39 (non-polar), instead of Lys39 (positively charged), was found in the snow leopard ( Fig. 2a , Supplementary Fig. S10 , Supplementary Table S44 ), indicating a significant change in charge that might alter protein function. This Met39 residue was replicated as a genetically fixed substitution in 14 additional snow leopards, whereas the ancestral Lys39 was monomorphic in a sampling of 28 individuals of Panthera and Neofelis (clouded leopard) ( Supplementary Table S45 , Supplementary Methods ). Naked mole rats have also adapted to hypoxia [22] in a different manner by having unique amino-acid changes in different positions of EGLN1 (Pro15, Arg17 and Arg36). Ile663 and Arg794 in EPAS1 are two additional snow leopard-specific changes ( Supplementary Fig. S11 ), and Arg794 was predicted to confer a functional change on the protein. Taken together, these EGLN1 and possibly EPAS1 variants are provocative candidates that may have contributed to the snow leopard’s acquisition of an alpine, high altitude ecological niche. 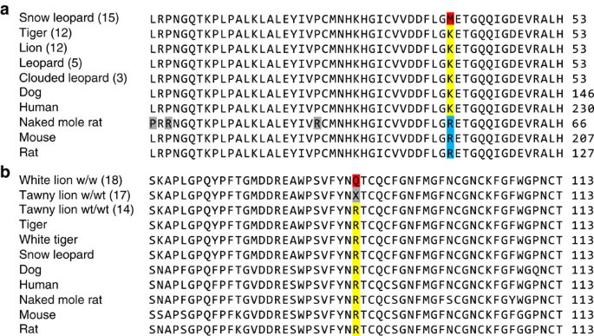Figure 2:EGLN1andTYRmutations related to hypoxia in snow leopard and white fur in white lion. (a) Alignment of mammalianEGLN1amino-acid sequences. Amino acids unique to the snow leopard (216th residue in humanEGLN1), naked mole rat and rodents are shown in red, grey and blue, respectively. The number of individuals genotyped in this study is listed in parentheses. (b) Alignment of mammalianTYRsequences. Amino-acid sequences unique to the white lion (87th residue in humanTYR) are shown in red, and tawny lion having heterozygous allele (G/A) are shown in grey; X represents amino acid of R/Q. The numbers in parentheses are number of individuals. ‘w’ denotes white type and ‘wt’ denotes wild type. Figure 2: EGLN1 and TYR mutations related to hypoxia in snow leopard and white fur in white lion. ( a ) Alignment of mammalian EGLN1 amino-acid sequences. Amino acids unique to the snow leopard (216th residue in human EGLN1 ), naked mole rat and rodents are shown in red, grey and blue, respectively. The number of individuals genotyped in this study is listed in parentheses. ( b ) Alignment of mammalian TYR sequences. Amino-acid sequences unique to the white lion (87th residue in human TYR ) are shown in red, and tawny lion having heterozygous allele (G/A) are shown in grey; X represents amino acid of R/Q. The numbers in parentheses are number of individuals. ‘w’ denotes white type and ‘wt’ denotes wild type. Full size image Tyrosinase ( TYR ) mutational variants cause white coat colour in the domestic cat [23] , and TYR mutations are related to human oculocutaneous albinism 1 (refs 24 , 25 ). The genetic basis of the white tiger with white fur and dark stripes is revealed as an amino-acid change (A477V) in the transporter protein SLC45A2 (ref. 26 ). Therefore, we examined the pigment-associated gene mutation in the white lion and found a unique nucleotide ( TYR 260G>A) and corresponding amino-acid change in the white lion ( Fig. 2b , Supplementary Fig. S12 ), causing the positively charged Arg87, located in the central domain of TYR , to be changed to uncharged Gln87. We verified the proposed candidate mutation ( TYR 260G>A) underlying the amino-acid change (R87Q) in the TYR gene sequence of 47 lions: 17 of white phenotype and 30 of wild phenotype, of which 11 were known to be carriers (heterozygotes) based on their pedigree, 14 of unknown genetic makeup, and 5 of wild phenotype from control populations where no white lions were found ( Supplementary Tables S46–S48 , Supplementary Methods ). The concordance between the expected and observed genotype was 100% for the candidate mutation TYR 260G>A. A second non-synonymous mutation ( TYR 176C>T), observed in a subset of animals, did not correlate with the expected genotype, and animals with this variant did not appear to be phenotypically different. Genomic comparison between the tiger and other mammals Although repeat characteristics can vary considerably among closely related species [27] , the tiger and cat genomes showed very similar repeat compositions (39.3% versus 39.2%, respectively), as well as ratios of repeat components, including tandem repeats and transposable elements ( Supplementary Fig. S13 ), suggesting a similar genome architecture between domestic cats and tigers. By contrast, for the great apes, the ratio of repeat components was considerably different between species, especially between human and orangutan, which diverged about 12 MYA [28] . Additionally, we estimated the evolutionarily conserved sequences (77 Mb, 3.2%), segmental duplication (11.2 Mb, 0.47%) and lineage-specific insertions and deletions in the tiger genome ( Supplementary Tables S49–S52 , Supplementary Methods ). To detect genome-wide structural differences, we aligned the tiger scaffolds to the cat genome using dog genome as a reference after masking repeats. A total of 571 of the 674 tiger scaffolds (length >20 kb, 99.6% of the total scaffold length) were aligned with the cat genome sequence, and as high as 98.8% of gene-coding regions and 98.3% (2.38 Gb) of conserved synteny blocks were shared by the tiger and cat genomes. We detected a rather high level of genomic synteny, containing six breaks with large-size chromosomal segmental rearrangement between the tiger and cat genomes ( Fig. 3 , Supplementary Fig. S14 , Supplementary Tables S53–S56 , Methods). These consisted of two inter- and four intra-chromosomal rearrangements. Divergence in genomic structure among closely related species is considered as a major factor underlying species diversification, as gene flow requires recombination in collinear chromosomes, and the reduction in recombination associated with chromosomal rearrangements results in a partial reproductive barrier [29] . These structural variations may be one of the important factors underlying species diversification among the felines. 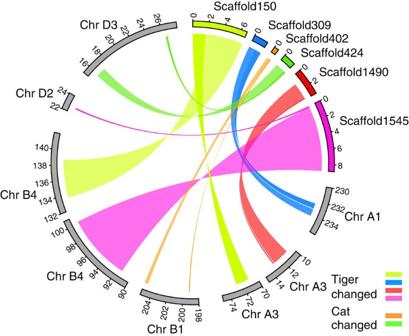Figure 3: Synteny blocks between tiger and cat genomes. Domestic cat chromosomes are shown as grey bars (in Mb scales). The other six color bars (in Mb scales) are tiger scaffolds with syntenic break between tiger and cat (2 inter- and 4 intra-chromosomal rearrangements). The tiger and cat rearrangements were detected using dog genome as an out-group. Figure 3: Synteny blocks between tiger and cat genomes. Domestic cat chromosomes are shown as grey bars (in Mb scales). The other six color bars (in Mb scales) are tiger scaffolds with syntenic break between tiger and cat (2 inter- and 4 intra-chromosomal rearrangements). The tiger and cat rearrangements were detected using dog genome as an out-group. Full size image The level of within-species genetic diversity, as measured by the rate of heterozygous SNVs, of the tiger (0.00049–0.00073) and lion (0.00048–0.00058) genomes was found to be similar to that of human (0.00066) ( Supplementary Table S57 , Supplementary Methods ). Interestingly, diversity of the snow leopard genome was nearly half that of the other Panthera species and slightly lower than that of the Tasmanian devil [30] , which is purported to display a low level of genetic diversity ( Fig. 4a ). We also estimated the occurrence of a marked bottleneck around the last glacial maximum 20 kyr ago (7–70 kyr) using a pairwise sequentially Markovian coalescent (PSMC) [31] model inference of tiger demographic history based on SNV distribution ( Fig. 4b , Supplementary Figs S15–S18 , Supplementary Tables S58 and S59 , Methods). A similar bottleneck was estimated a bit earlier (72–108 kyr) based on mitochondrial DNA coalescence [1] . White lion (0.00048) and domestic cat (0.00012) have both undergone multiple rounds of close inbreeding during breed development and therefore would display lower SNV diversity bias as a consequence. Therefore, we investigated the genetic diversity of Panthera using the rate of heterozygous SNVs and confirmed that the genetic diversity within a single individual coincided with that deduced from mitochondrial sequences of several individuals [30] . 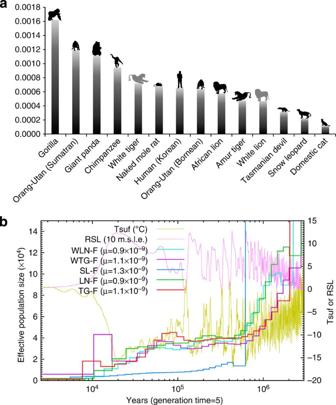Figure 4: Genetic diversity and population size history inPantheraspecies. (a) Rate of heterozygous SNVs inPantheraspecies. The heterozygous SNVs rates (yaxis) were calculated by dividing the total number of heterozygous SNVs by genome size. Individuals that are white colored in nature (white tiger and white lion) are shown in grey. Tigers, lions, cat, gorilla, giant panda, chimpanzee and naked mole rat are captive bred. Snow leopard, orang-utans and Tasmanian devil are wild caught individuals. (b) Estimated big cat population sizes and climate history from 2.5 kyr BP to 3 Myr BP. Tsuf, atmospheric surface air temperature; RSL, relative sea level; 10 m.s.l.e., 10 m sea level equivalent; TG, Amur tiger; LN, African lion; SL, snow leopard; WTG, white tiger; WLN, white African lion. ‘F’ after the species abbreviation means the data were generated from comparison with Felis_catus-6.2 as a reference genome in SNV calling. Figure 4: Genetic diversity and population size history in Panthera species. ( a ) Rate of heterozygous SNVs in Panthera species. The heterozygous SNVs rates ( y axis) were calculated by dividing the total number of heterozygous SNVs by genome size. Individuals that are white colored in nature (white tiger and white lion) are shown in grey. Tigers, lions, cat, gorilla, giant panda, chimpanzee and naked mole rat are captive bred. Snow leopard, orang-utans and Tasmanian devil are wild caught individuals. ( b ) Estimated big cat population sizes and climate history from 2.5 kyr BP to 3 Myr BP. Tsuf, atmospheric surface air temperature; RSL, relative sea level; 10 m.s.l.e., 10 m sea level equivalent; TG, Amur tiger; LN, African lion; SL, snow leopard; WTG, white tiger; WLN, white African lion. ‘F’ after the species abbreviation means the data were generated from comparison with Felis_catus-6.2 as a reference genome in SNV calling. Full size image The Amur tiger genome is the first reference genome sequenced from the Panthera lineage and the second from the Felidae species. For comparative genomic analyses of big cats, we additionally sequenced four other Panthera genomes and tried to predict possible big cats’ molecular adaptations consistent with the obligatory meat eating and muscle strength of the predatory Panthera lineage. The tiger and cat genomes showed unexpectedly similar repeat compositions and high genomic synteny, and these indicated strong genomic conservation in Felidae. These results could be supported by the recency of the 37 species-Felidae radiation (<11 MYA) [15] and well-known hybridizations in captivity among subspecies in Felidae lineage such as liger and tigon. By contrast, the ratio of repeat components for the great apes was considerably different among species, especially between human and orang-utan [28] , which diverged about the same time as felines. The breaks in synteny that we observed are likely occasional rare sporadic exchanges that accumulated over this short period (<11 MYA) of evolutionary time. The paucity of exchanges across the mammalian radiations (by contrast to more reshuffled species such as Canidae, Gibbons, Ursidae and New World monkeys) is a hallmark of evolutionary constraints. Many whole-reference genome studies used few close species genomes that can be directly compared with the reference genome constructed. Although we did not have the resources to construct lion and leopard reference genomes, and hence were not able to show all the structural variations on the genomes, our ‘close species comparative genomics’ approach, utilizing at least one reference species, heralds a new level of genome studies. It is because those very close Panthera species have distinct species-specific and readily identifiable phenotypes that can be associated quickly to mutations by comparing the homologous genes of interest as shown in the fur colouring (white lion) and high-altitude adaptation (snow leopard). If sufficiently distinct phenotypes are biologically curated, genetic mutations causing species specificity can be systematically detected using next generation sequencing. Once such candidate genetic mutations are confirmed in the set of species genomes, experimental validations can be carried out, as in the additional 47 lion samples here, for targeted genes. This genetic variation comparison using whole genomes among species and subspecies can thus provide valuable insight and information for the whole family’s conservation. Our data from tigers, lions and snow leopard can provide a rich and diverse genome resource that could be used in future studies of conservation and population genomics so that the genetic underpinnings of local adaptation and potential inbreeding and/or outbreeding [10] in wild and captive populations can be illuminated and thereby help ensure the future survival of these majestic species. Genome sequence assembly and annotation The blood samples used for genome sequencing were acquired from the Everland Zoo of Korea (Amur tiger, white Bengal tiger, African lion and white African lion) following the Everland Zoo (Korea) ethical guidelines and procedures, and a muscle sample was obtained from a Mongolian snow leopard carcass preserved in the Conservation Genome Resource Bank for Korean Wildlife, Seoul National University. No animals were killed or captured as a result of this study. Libraries for the Amur tiger genome were constructed at BGI, Shenzhen, and the insert sizes of the libraries were 170 bp, 500 bp, 800 bp, 2 kb, 5 kb, 10 kb and 20 kb. The libraries were sequenced using HiSeq2000. Other big cat genomes were sequenced at Theragen BiO Institute (TBI), Korea, using HiSeq2000 with read and insert lengths of ~90 bp and ~400 bp, respectively. The corrected reads were used to complete the genome assembly using SOAPdenovo [13] . First, the short insert size library (170 bp, 500 bp and 800 bp) data were used to construct a de Bruijn graph. Second, all reads were realigned with the contig sequences. The amount of shared paired-end relationships between pairs of contigs were calculated and weighted with the rate of consistent and conflicting paired ends, before constructing the scaffolds step by step from the short insert size paired ends to the long distant paired ends. Third, the gaps between the constructed scaffolds were closed using the paired-end information to retrieve read pairs where one end mapped to a unique contig while the other was located in the gap region. The Amur tiger genes were predicted using three approaches. First, de novo prediction was performed using the repeat-masked genome using AUGUSTUS (version 2.5.5) [32] and GENSCAN (version 1.0) [33] . Second, homologous proteins in other species were mapped to the genome using tBLASTn (Blast 2.2.23) [34] with an E-value cutoff of 1E-5. The aligned sequence and its query protein were then filtered and passed to GeneWise (version 2.2.0) [35] to search for accurately spliced alignments. Third, cat EST and full-length cDNA sequences (from UCSC) were aligned to the genome using BLAT [36] to generate spliced alignments. For EST results, spliced alignments were linked according to overlap using PASA [37] . Source evidence generated from the three approaches was integrated with GLEAN [38] to produce a consensus gene set. Then, the Amur tiger genome sequence was aligned to two well-assembled and annotated genomes (human and domestic cat) using LASTZ (version 1.02). Finally, mapped results yielding information on homologous proteins were filtered by syntenic blocks of genome sequences. We also predicted the domestic cat (Felis_catus-6.2) gene set, because the gene set of the cat genome is preliminary. Orthologous gene families A comparative analysis was used to examine the rate of protein evolution and the conservation of gene repertoires among orthologs in the genomes of the Amur tiger, dog, human, mouse, giant panda, domestic cat (Felis_catus-6.2) and opossum. We used the TreeFam methodology [39] to define a gene family as a group of genes that descended from a single gene in the last common ancestor of a considered species. We assigned a connection (edge) between two nodes (genes) if more than 1/3 of the region was aligned to both genes. An H-score (minimum edge weight) that ranged from 0 to 100 was used to weigh the similarity (edge). For two genes, G1 and G2, the H-score was defined as score (G1G2)/max (score (G1G1), score (G2G2)), where the score shown is the BLAST raw score. Gene families were extracted by clustering using Hcluster_sg. We used the average distance for the hierarchical clustering algorithm, requiring the H-score to be larger than five, and the minimum edge density (total number of edges/theoretical number of edges) to be larger than 1/3. The clustering for a gene family would also stop if it already had one or more of the out-group genes. We determined the expansion and contraction of the orthologous protein families among seven mammalian species (tiger, cat (Felis_catus-6.2), dog, human, mouse, giant panda and opossum) using CAFÉ 2.2 (ref. 40 ) with 0.001080 of lambda option. GO of all tiger genes was annotated by InterPro. A χ 2 test followed by a Fisher’s exact test ( P ≤0.01) were used to test for over-represented functional categories among expanded genes and ‘genome background’ genes; Fisher’s exact test was used when any expected value of count was below 5, which would have make the χ 2 test inaccurate [41] . Gene evolution We investigated Panthera lineage-specific amino-acid changes by comparison with the known genes from the human, dog and mouse (from the Ensembl 69 release). We used lion and snow leopard gene sets by mapping reads to the tiger scaffolds and substituting SNVs. Artifacts from the multiple sequence alignment (ClustalW2 [42] ) limitations were removed by filtering option with ≥1/2 of coverage and ≥of well-matched amino acids (consensus string is ‘*’, ‘:’ or ‘.’). To detect tiger genes evolving under positive selection, we used conserved genome synteny methodology [19] to establish a high-confidence orthologous gene set. Briefly, whole-genome multiple alignments were performed between human (hg19) and other species (cat (Felis_catus-6.2), dog (CanFam2.0), mouse (mm9) and panda (ailMel1) genomes) by the LASTZ alignment pipeline. We collected all the human protein-coding genes from RefSeq [43] , KnownGene [44] and VEGA [45] , and mapped them to the other species via the syntenic regions. We then filtered the resulting blocks with rigorous conditions to get large-scale synteny of high-alignment quality, and a conservation of exon–intron structure. Finally, we found 7,415 1:1 high-quality ortholog genes to analyse, most of which also correspond to genes in the panda, dog and mouse genomes. Then, we aligned ortholog genes by PRANK [46] and used the optimized branch-site model of PAML (version 4.5) and likelihood ratio tests (LRTs) ( P ≤0.05). A GO annotation download from Ensembl was used to assign GO categories to 7,415 orthologs. A χ 2 test followed by a Fisher’s exact test ( P ≤0.01) were used to test for over-represented functional categories among positively selected genes; a Fisher’s exact test was used when any expected value of count was below 5, which would have made the χ 2 test inaccurate [41] . We also used an approach based on Ka / Ks [47] , [48] to identify GO categories significantly above or below average in the tiger genome. The Ka and Ks rates are estimated by PAML from all aligned bases with a quality score >20 in orthologs, using the F3 × 4 codon frequency model and the REV substitution matrix. To determine whether the GO categories are evolving under significantly high constraints, we repeated this procedure 10,000 times on the same data set after randomly permuting the GO annotations. Then, we acquired the GO categories if the P -value was less than 0.05. Chromosomal rearrangement Among the alignment data generated from SyMAP [49] , when one scaffold happened to be mapped to several physically distant cat (Felis_catus-6.2) chromosomal locations, they were considered to be inter- or intra-chromosomal rearrangement events of the Amur tiger genome relative to the cat genome. The species (tiger and domestic cat)-specific genomic rearrangements were also analysed. We performed the dog versus tiger and cat versus tiger whole-genome pair-wise alignments using LASTZ software on the repeat-masked genomes. Using these methods, we identified clusters of unique alignments with well-defined order and orientation. There was a total of 18 chromosomal rearrangement (12 inter- and 6 intra-chromosomal rearrangements) overlaps when the results from SyMAP and LASTZ were integrated by comparing syntenic break positions. As the tiger assembly was generally fragmented, we carefully validated the 18 syntenic breaks to examine the assembly integrity by aligning long insert mate-pair libraries (2 kb, 5 kb, 10 kb and 20 kb) to the tiger scaffolds. Finally, we reported six putative chromosomal rearrangements (two inter- and four intra-chromosomal rearrangements) between the tiger and cat. All six rearrangements were validated by long-range PCR experiments followed by the Sanger sequencing method. Demographic history The history of population size helps to develop insights into evolution. Based on the pairwise sequentially Markovian coalescent model (PSMC) [31] , we inferred detailed population size histories of Amur tiger (TG), African lion (LN), snow leopard (SL), white tiger (WTG) and white lion (WLN). Using SNV data sets scanned with all the big cat sequencing reads mapped to Felis_catus-6.2, the consensus sequences of each big cat were constructed and then divided into non-overlapping 100-bp bins marked as homozygous or heterozygous. The resultant bin sequences for their sex chromosomal parts were removed, and then they were taken as the input of the PSMC estimation. To test the estimation accuracy, bootstrapping was performed by randomly resampling 100 sequences from the original sequences. Using the neutral mutation rates, the raw PSMC outputs were scaled to time and population sizes. We obtained atmospheric surface air temperature and global relative sea level data of the past 3 million years [50] . Accession codes: The Amur tiger whole-genome shotgun project has been deposited at DDBJ/EMBL/GenBank under the accession number ATCQ00000000. The version described in this paper is the first version, ATCQ01000000. Raw DNA and RNA sequencing reads have been submitted to the NCBI Sequence Read Archive database ( SRA074975 , SRA091968 ). How to cite this article: Cho, Y. S. et al. The tiger genome and comparative analysis with lion and snow leopard genomes. Nat. Commun. 4:2433 doi: 10.1038/ncomms3433 (2013).